Kinship reduces alloparental care in cooperative cichlids where helpers pay-to-stay Alloparental brood care, where individuals help raising the offspring of others, is generally believed to be favoured by high degrees of relatedness between helpers and recipients. Here we show that in cooperatively breeding cichlids, unrelated subordinate females provide more alloparental care than related ones when kinship between dominant and subordinate group members is experimentally manipulated. In addition, unrelated helpers increased alloparental care after we simulated egg cannibalism by helpers, an effect not shown by related helpers. By supporting predictions of pay-to-stay theory, these results suggest that in Neolamprologus pulcher , reciprocal commodity trading is important for the decision of subordinates to invest in care of the dominants’ offspring. Kinship is assumed to promote the evolution of cooperation and sociality in animals [1] , [2] , [3] . Subordinate, non-reproductive members of social groups can gain indirect fitness benefits if they are related to the dominant breeders and distribute their help according to kinship [4] . Among vertebrates, evidence for the importance of indirect fitness benefits exists for some bird species, for example, Seychelles warblers [5] , Long-tailed tits [6] , [7] and Bell miners [8] , [9] . However, several studies did not find kinship effects on helping behaviour as predicted by kin-selection theory (in mammals [10] ; fish [11] ; birds [12] ; insects [13] ) and substantial help is sometimes shown by unrelated individuals [9] , [14] , [15] , [16] . Furthermore, unrelated helpers exist in all aforementioned systems. Together, this suggests the existence of direct fitness benefits to helpers [17] , [18] . Such benefits were experimentally demonstrated in cooperatively breeding vertebrates [19] and can explain cooperative brood care also in some primitively eusocial insects [20] . Direct fitness benefits to subordinates can be accrued for instance by group augmentation, if the survival of group members increases with group size [21] and the costs of helping behaviour are outweighed by the benefits of a magnified group size [22] , [23] , [24] , [25] . In addition, subordinates may benefit from group membership without group augmentation, for instance because this provides them with access to limited resources or enhances protection from predators [19] . If dominant group members incur costs from the presence of subordinates, for example through competition for resources or for reproduction, they may enforce help from subordinates (for example, to raise the dominants’ offspring) in order to compensate for these costs. If subordinates consequently ‘pay-to-stay’ in the group, this resembles the exchange of services in different commodities [26] . Such helping by demand, or through coercion, may apply particularly when relatedness between dominants and subordinates is low, the presence of subordinates inflicts costs on dominants, dispersal and survival outside of groups and independent breeding by subordinates are constrained, and individuals are generally long-lived [27] , [28] . However, if pay-to-stay is the ultimate cause of helping behaviour, subordinates should only compensate for the costs they inflict on dominants, and dominants will gain no net fitness benefits from the presence and help of subordinates [28] . Furthermore, if subordinates help because they are coerced to do so by dominants, the conventional predictions of kin-selection theory are reversed: in this case related individuals are expected to provide less help than unrelated ones [27] . Hence, the pay-to-stay hypothesis takes kinship effects into account [26] , [27] , [28] and generates testable predictions about the effect of relatedness on helping behaviour. Hitherto, these predictions have been rarely scrutinized empirically, despite evidence for this form of reciprocity in a wide range of vertebrates [15] , [29] , [30] , [31] , [32] . It is important to note that the three mentioned mechanisms, kin-selection, group augmentation and helping by coercion are not mutually exclusive and may operate in a social system in conjunction. In essence they constitute different means how helping can afford net inclusive fitness benefits to subordinate group members. It is hitherto largely unexplored how behaviour in cooperative societies is shaped by the interplay of these mechanisms, if groups consist of a mixture of related and unrelated individuals [33] . It is possible that potential conflict of interests between dominant and subordinate members within such groups of cooperative breeders can be resolved by two mechanisms acting in parallel. First, unrelated subordinates are coerced to provide help to dominants in order to compensate for costs they incur on the latter, that is, they pay to be allowed to stay in the group. Second, subordinates that are related to dominants profit from helping the latter by indirect fitness benefits, and hence helping does not need to be coerced and no rent needs to be paid by them. If mainly kin-selected benefits are important for behavioural and reproductive decisions of the group members, it is expected that relatedness between breeders and helpers would yield lower eviction rates of subordinates and enhanced alloparental brood care provided by the subordinate to the dominant female’s brood and vice versa. Accordingly, both dominants and subordinates should invest more in offspring production, yielding a higher reproductive success in kin compared with non-kin groups. If in contrast, dominants force subordinates to provide help, such as assumed by pay-to-stay models, unrelated subordinate females should provide more alloparental brood care than related ones, and unrelated subordinates should be evicted more readily by dominants if they do not compensate for the lack of kinship by increased helping levels (that is, payment). If such compensation occurs, however, similar eviction rates of related and unrelated subordinates might be expected in case helping depends on coercion [28] . Furthermore, if subordinates breed in the territory of dominants [34] , alloparental brood care should not be reciprocated by the dominant female [35] in a pay-to-stay scenario, and dominant female fitness should be independent of relatedness to subordinates, as helper payment may only compensate for imposed costs and not provide net fitness benefits to dominants [28] . Finally, if helping is triggered by coercion and if unrelated subordinates need to compensate for imposing costs on dominants [27] , [28] , they should increase their investment in alloparental brood care behaviour if these costs to dominants are experimentally raised; in contrast, such increased cost compensation should be weaker or absent in related subordinates. When testing predictions concerning the mechanism maintaining helping behaviour in cooperative breeders, it is important to scrutinize effects on alloparental brood care, because this involves temporary fitness costs [36] , [37] to subordinates without generating immediate shared benefits. Other helping behaviours such as predator defence and territory maintenance might also serve immediate direct fitness benefits to subordinates (that is, being ‘selfish’ [38] , [39] ), which is not the case with alloparental care. Alternatively or in addition to the operation of a pay-to-stay mechanism, alloparental care could yield direct fitness benefits to helpers by group augmentation. It is, therefore, also important to control for potential effects of group augmentation benefits when aiming to unravel the relative importance of relatedness and commodity trading for fitness effects of alloparental care. Here our aim is to test the relative importance of kin-selection and coerced helping experimentally using the cooperatively breeding cichlid N. pulcher as a model (see methods section for a description of the organism). Specifically, we test the crucial predictions of kin-selection and pay-to-stay hypotheses with regard to the effect of relatedness between helpers and beneficiaries. We experimentally manipulated kinship among female group members to study potential effects on female reproduction and alloparental brood care, both by dominant and subordinate females. We assembled groups of a pair and a female subordinate helper, where the dominant and subordinate females were either related (‘kin’ treatment: females were full sisters or mother–daughter; relatedness r =0.5), or unrelated (‘non-kin’ treatment; r =0.0). We test predictions derived from pay-to-stay and conventional kin-selection theory regarding eviction probability, reproductive participation and alloparental brood care by the female group members [1] , [21] , [26] , [27] , [28] , while controlling for potential benefits of group augmentation. Additionally, we manipulated the dominants’ perceived costs of a subordinate’s presence in the group by experimentally inducing perceived egg cannibalism of the latter in groups with related and unrelated subordinates (below referred to as ‘compensation experiment’). We found that unrelated subordinate females provide more alloparental care than related ones and that unrelated helpers increased alloparental care after we simulated egg cannibalism by helpers, an effect not shown by related helpers. These results are consistent with models of helping by coercion such as pay-to-stay and suggest that N. pulcher subordinates trade alloparental brood care against being tolerated in the territory. Eviction of subordinates In the cooperatively breeding cichlid N. pulcher ( Fig. 1a ) female kinship did not influence whether the subordinate was accepted, tolerated or evicted (see inset Fig. 2a for the frequencies; ordinal regression: LR χ 2 =2.8, df=2, P =0.24, N =69). Only the size difference between females affected eviction ( Fig. 2a ; ordinal regression: χ 2 =4.9, coefficient=−0.05±0.02, P =0.027, N =69). Subordinate eviction usually happened in the first days after release of the pair ( N =23, median day of eviction=3, Range: day 0–day 41) and again, the latency to eviction did not depend on female kinship ( Fig. 2b , general linear model (GLM), effect of kinship: Wald χ 2 =0.6, df=1, P =0.45). 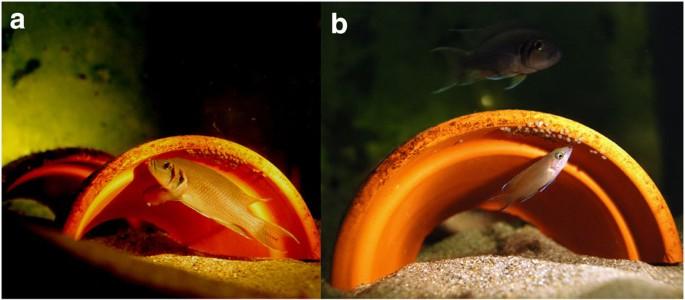Figure 1: An experimentally createdN. pulchergroup caring for the dominant female‘s brood. (a) The dominant female cleans a clutch attached to the breeding cavity with gentle micronips, while the subordinate female is submissively touching the dominant female’s throat with the tail fin. (b) The subordinate female cleans the eggs laid by the dominant female, providing alloparental brood care. (Photos: M.Z.) Figure 1: An experimentally created N. pulcher group caring for the dominant female‘s brood. ( a ) The dominant female cleans a clutch attached to the breeding cavity with gentle micronips, while the subordinate female is submissively touching the dominant female’s throat with the tail fin. ( b ) The subordinate female cleans the eggs laid by the dominant female, providing alloparental brood care. (Photos: M.Z.) 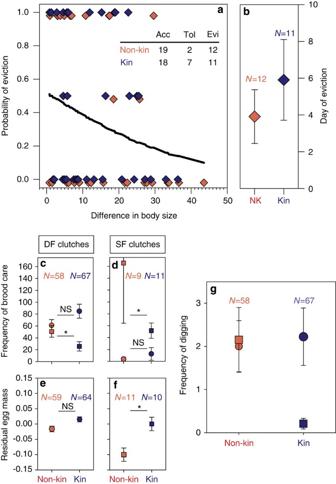Figure 2: Subordinate eviction and alloparental brood care. (a) Subordinates’ probability of eviction decreased significantly with the difference in female size (dominant female body size—subordinate female body size), but did not depend on female kinship (blue filling: kin, red filling: non-kin). Inset shows number of subordinates accepted (Acc), tolerated (Tol) and evicted (Evi), depending on kinship. The line shows the predicted probability of eviction from the ordinal regression. For clarity, blue and red symbols were slightly off-set to avoid overlap. (b) Day of eviction since release (latency in days) of subordinate females did not depend on kinship (NK, non-kin groups; kin, kin groups). (c) Care provided to dominant female (DF) clutches and (d) subordinate female (SF) clutches per treatment (blue filled symbols: kin, red filled symbols: non-kin) and the group member (dominant females: circles; subordinate females: squares). Unrelated subordinate provided significantly more alloparental brood care to dominant female clutches than related ones. This did however not affect the maternal investment in brood care of dominant females. Subordinate clutches received very low levels of alloparental care from the dominant females, and maternal levels of brood care in subordinate females were higher in the non-kin groups. (e) Dominant and (f) subordinate female residual single-egg mass (corrected for intercept and female body size effects). Subordinate females laid heavier eggs in the kin groups, whereas egg mass in dominant female clutches did not differ between treatments. (g) Sand removal when dominant female clutches were present per kinship treatment (red filled symbols: non-kin, blue filled symbols: kin) and the group member (dominant females: circles; subordinate females: squares). Unrelated subordinate females exhibited higher levels of sand removals than related females. Dominant females did not differ between the treatments in their investment in digging. Depicted are means±s.e.m. SeeTables 1,2,3,4for model details. The upper error bar of the values of non-kin subordinate females in paneldis cutoff in favour of a generally greater resolution of values on the ordinate. Sample sizes are indicated in the graph. Asterisk denotes significance. Full size image Figure 2: Subordinate eviction and alloparental brood care. ( a ) Subordinates’ probability of eviction decreased significantly with the difference in female size (dominant female body size—subordinate female body size), but did not depend on female kinship (blue filling: kin, red filling: non-kin). Inset shows number of subordinates accepted (Acc), tolerated (Tol) and evicted (Evi), depending on kinship. The line shows the predicted probability of eviction from the ordinal regression. For clarity, blue and red symbols were slightly off-set to avoid overlap. ( b ) Day of eviction since release (latency in days) of subordinate females did not depend on kinship (NK, non-kin groups; kin, kin groups). ( c ) Care provided to dominant female (DF) clutches and ( d ) subordinate female (SF) clutches per treatment (blue filled symbols: kin, red filled symbols: non-kin) and the group member (dominant females: circles; subordinate females: squares). Unrelated subordinate provided significantly more alloparental brood care to dominant female clutches than related ones. This did however not affect the maternal investment in brood care of dominant females. Subordinate clutches received very low levels of alloparental care from the dominant females, and maternal levels of brood care in subordinate females were higher in the non-kin groups. ( e ) Dominant and ( f ) subordinate female residual single-egg mass (corrected for intercept and female body size effects). Subordinate females laid heavier eggs in the kin groups, whereas egg mass in dominant female clutches did not differ between treatments. ( g ) Sand removal when dominant female clutches were present per kinship treatment (red filled symbols: non-kin, blue filled symbols: kin) and the group member (dominant females: circles; subordinate females: squares). Unrelated subordinate females exhibited higher levels of sand removals than related females. Dominant females did not differ between the treatments in their investment in digging. Depicted are means±s.e.m. See Tables 1 , 2 , 3 , 4 for model details. The upper error bar of the values of non-kin subordinate females in panel d is cutoff in favour of a generally greater resolution of values on the ordinate. Sample sizes are indicated in the graph. Asterisk denotes significance. Full size image Alloparental brood care Against predictions from helping to accrue kin selected, indirect benefits, but confirming predictions from helping due to coercion, subordinate females provided significantly less alloparental brood care in the kin treatment than in the non‐kin treatment ( Fig. 2c , Table 1 ). Increasing clutch size had positive effects on the amount of alloparental brood care provided, whereas increasing body size of the subordinate females had the opposite effect ( Table 1 ). Similarly to direct brood care, unrelated subordinates provided also more indirect brood care than related subordinates by removing sand from the breeding cavity when eggs were present ( Fig. 2g , Table 2 ). In contrast to subordinates, the digging effort of dominant females did not differ between the two treatments ( Fig. 2g , Table 2 ). Table 1 Effects of female kinship on brood care. Full size table Table 2 Effects of female kinship on removal of sand. Full size table In 18 of 69 replicates the subordinate females produced a total of 28 clutches, which allowed comparing maternal and alloparental care of both females. Kinship did not affect maternal ( Fig. 2c ) and alloparental brood care ( Fig. 2d ) provided by the dominant female ( Table 1 ). The level of alloparental brood care provided by the dominant female was very low ( Fig. 2d ) compared with the level of alloparental brood care provided by the subordinate female ( Fig. 2c ). Kinship apparently affected the brood care behaviour of the subordinate females: they provided significantly more maternal brood care in the non-kin treatment than in the kin treatment ( Fig. 2d , Table 1 ). However, this result is characterized by large variance ( Fig. 2d ) caused by an exceptionally high value of one subordinate female, and hence it should to be treated as tentative. 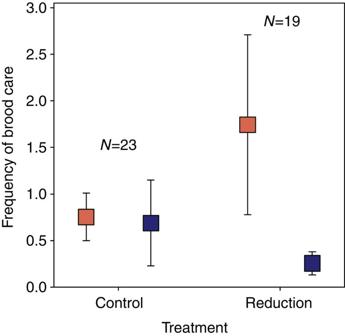Figure 3: Compensation experiment. Alloparental brood care from related (blue squares) and unrelated (red squares) subordinate females provided to dominant females' clutches after the simulated egg cannibalism (Reduction) or after the control manipulation (Control), controlled for clutch size. The interaction relatedness × treatment (Reduction/Control) is significant, indicating that unrelated subordinate females increased their investment in alloparental brood care compared with related subordinates when the clutch size was reduced to simulate egg cannibalism. Depicted are means±s.e.m., sample sizes are indicated in the graph. SeeTable 3for model details. In the ‘compensation experiment’, unrelated subordinate females increased their investment in alloparental brood care compared with related subordinates when the clutch size was reduced to simulate egg cannibalism, as revealed by the significant interaction of kinship and treatment, when controlling for the effect of brood size (smaller clutches generally received less care; Table 3 ; Fig. 3 ). Furthermore, there was a body size effect, with small female subordinates providing more care than larger ones ( Table 3 ). Table 3 Alloparental brood care after clutch manipulation. Full size table Figure 3: Compensation experiment. Alloparental brood care from related (blue squares) and unrelated (red squares) subordinate females provided to dominant females' clutches after the simulated egg cannibalism (Reduction) or after the control manipulation (Control), controlled for clutch size. The interaction relatedness × treatment (Reduction/Control) is significant, indicating that unrelated subordinate females increased their investment in alloparental brood care compared with related subordinates when the clutch size was reduced to simulate egg cannibalism. Depicted are means±s.e.m., sample sizes are indicated in the graph. See Table 3 for model details. Full size image Female reproduction Dominant female reproduction was not affected by kinship ( Table 4 , Fig. 2e , Supplementary Fig. S3a,c ; corrected for effects of female body size and duration of the experiment). The number of clutches produced by the subordinate female and clutch size was also not affected by kinship ( Table 4 , Supplementary Fig. S3b,d ), but egg mass of subordinate females was affected by kinship ( Fig. 2f ): related subordinate females produced significantly larger eggs than unrelated subordinate females. Furthermore, larger subordinates produced significantly more clutches, containing more and heavier eggs then smaller subordinates ( Table 4 ). In dominant females a similar effect of body size appeared only for clutch size and tentatively for egg mass, whereas there was no effect on the number of clutches produced ( Table 4 ). Table 4 Effects of female kinship and female body length on female reproduction. Full size table Social behaviour The aggression of dominant females towards female subordinates ( Supplementary Fig. S2a,b ), the submissive behaviour of subordinate females towards dominant females ( Supplementary Fig. S2c,d ) and the breeding shelter visits of subordinates ( Supplementary Fig. S2e,f ) were all unaffected by kinship ( Supplementary Table S1 ), also when corrected for female size. The difference between female sizes in a group, however, predicted the number of breeding shelter visits of subordinate females. Large differences in body size between females resulted in more breeding shelter visits of subordinate females ( Supplementary Table S1 ). If anything, related subordinates tended to make more breeding shelter visits than unrelated ones ( Supplementary Fig. S2f ), and this coincided with more aggression received from the dominant female ( Supplementary Fig. S2b ) and a concomitant tendency of related subordinates to exhibit more submission towards dominant females than unrelated ones ( Supplementary Fig. S2d ). Eviction rates did not differ between related and unrelated subordinates, which is consistent with predictions from helping by coercion and pay-to-stay models [26] , [27] , [28] in the case where unrelated subordinates provide more brood care than related ones. The extra effort of non-kin may compensate for the lack of indirect fitness benefits to dominants when they tolerate unrelated subordinate group members. In contrast, kin-selection theory predicts that relatedness enhances tolerance [1] , which was clearly not the case ( Table 5 ). Table 5 Predictions evaluated in this study. Full size table The only significant predictor for eviction probability was the size difference between the dominant and subordinate females. As expected, the size difference between the dominant male and the subordinate female did not affect helper eviction. This suggests that eviction is partly associated with reproductive competition between dominant and subordinate females, which has been shown to increase when the two females are of similar size [40] . The majority of evictions occurred very fast (that is, the median time to eviction was only 4–6 days from start of experiment), and hence usually happened before the first breeding attempt of the pair. Therefore, the helpers evicted in this experiment could not increase the likelihood of being tolerated by showing direct brood care behaviour. As predicted by the pay-to-stay hypothesis [26] , [27] , [28] , unrelated subordinate female helpers provided more alloparental brood care than related ones and also participated more in digging out the brood cavity when eggs were present ( Fig. 2c ). Especially the latter behaviour has been shown to involve substantial energetic costs, as it results in a more than sixfold increase of routine metabolic rate [36] , [37] . Thus, unrelated females appear to invest more into costly alloparental brood care, which refutes the hypothesis that indirect fitness benefits are responsible for maintaining helping behaviour in these cooperatively breeding vertebrates. Clutches produced by the subordinate females received little alloparental care from the dominant female, which suggests that alloparental care of subordinates is not reciprocated by dominant females. Thus, reciprocal exchange of the same commodity [41] , resembling for instance a tit-for-tat paradigm, appears not to be important for brood care decisions of N. pulcher females [35] . The patterns of alloparental brood care we found cannot be explained solely by kin-selection [1] or by group augmentation models [21] , without involving coercive mechanisms (see Table 5 for summary). Rather, the cooperative behaviour of N. pulcher helpers seems to reflect a trading of different commodities between dominants and subordinates, where the access to vital resources within a safe territory is traded against participation in brood care and other duties. Experimental clutch reduction led to a relative increase in alloparental brood care of unrelated subordinate females compared with related subordinate females, suggesting that compensation as predicted by the pay-to-stay hypothesis [26] , [27] , [28] might explain the alloparental brood care effort of unrelated females. In contrast, potential conflicts of interest between dominant females and related subordinates might be resolved primarily by indirect fitness benefits to one or both parties; for instance, tolerating a daughter or sister may raise the inclusive fitness of a dominant female even if her presence incurs some costs. This illustrates that kin-selection and helping by coercion can act side by side within a species to select for the same altruistic behaviour in related and unrelated subordinates of cooperatively breeding vertebrates, even if for different reasons. As unrelated helpers exist in many cooperative breeders, our results might suggest that apart from kin-selection, direct fitness benefits of alloparental care may be more important than previously thought (see refs 9 , 15 , 17 , 20 ). Previous studies have provided additional support that N. pulcher helpers pay-to-stay in a territory of dominants. Large helpers of this species are often unrelated to the dominant breeders [16] , [42] , which calls for mechanisms other than kin-selection to explain the cooperative effort of subordinates. Individuals prevented from helping by removal were attacked by other helpers upon their return, which might suggest punishment [43] but could also reflect competition for dominance [39] . Helpers prevented from helping to defend the territory against intruders subsequently showed increased levels of cooperative defence, but experienced unchanged aggression levels [44] . In response to the experimental manipulation, individual helpers increased either cooperative defence or submissive behaviour, suggesting that cooperative defence may serve an appeasement function similarly to submissive displays [44] . Likewise, in another experiment large helpers responded to dominants’ aggression with submissiveness when competition was low, but instead with increased defence effort when the pressure on the territory was high [45] . Large helpers reduced cooperative territory maintenance (digging) in their home territories when experimentally provided with alternative breeding options elsewhere [46] . When the risk was experimentally increased by exposing natural groups to a piscivore predator, all helpers increased cooperative territory defence and maintenance, and large helpers in particular increased their defence effort per aggression received from dominants [38] . Finally, subordinates increased defence when experimentally exposed to egg predators that do not pose a physical threat to the helpers themselves [47] . Some of this previously reported evidence for pay-to-stay might alternatively be explained by direct fitness benefits to helpers without involving coercion by dominants, because territory defence and maintenance might generate immediate shared benefits [17] , [39] . Therefore, the cooperative behaviour experimentally elicited in this study is of crucial importance for a test of the pay-to-stay hypothesis, as alloparental egg-care does not provide immediate fitness benefits to unrelated helpers, whereas it involves clear costs [36] , [37] . As this helping effort is hence altruistic, it can be selected for only if helpers receive other fitness benefits in return, which result from the tolerance in a safe territory that provides them with access to vital resources such as shelter and protection [19] , [29] , [48] , and opportunities to share in reproduction [49] , [50] . In a previous study of kinship effects on the behaviour of N. pulcher group members in the laboratory, helpers related to both dominants showed less work effort (sum of shelter visits and territory defence) than unrelated helpers [16] , which is consistent with our results. In the field this effect applied only with regard to the relatedness between helpers and male breeders, while an opposite kinship effect emerged regarding relatedness between helpers and female breeders [16] . In contrast, a recent experimental laboratory study did not detect an influence of relatedness on territory maintenance or defence of helpers [11] . It should be noted, however, that in these studies direct brood care (that is, egg cleaning and fanning) could not be measured and potential effects of subordinate reproduction were not considered, which can strongly affect subordinate helping effort [35] , [49] . Potential effects of relatedness on alloparental brood care have generally received much attention [4] . However, in most vertebrates relatedness of group members cannot be experimentally manipulated. In the only study so far where this has been done, subordinate long-tailed tits helped more when related to beneficiaries than when unrelated, as predicted by kin-selection theory [6] without involving coercion, which is an opposite effect to our results reported here. Recently it has been suggested that reciprocal exchange of resources or services is rare in nature, if occurring at all, and that reciprocity in animal societies can be explained usually by intra-specific mutualism or manipulation [17] . To distinguish reciprocity from other forms of cooperation it is important to critically evaluate if social interactions involve temporary fitness costs, resemble the exchange of services or resources, generate immediate shared benefits, and happen regularly between unrelated individuals [17] . These conditions have been experimentally demonstrated in our study species, where temporary fitness costs of helping are caused by the increased energy expenditure of different helping behaviours [36] , [37] , which can affect growth [19] . Access to resources in a safe territory is traded against help in defence against competitors [44] and immediate shared benefits to the group members can be generated by cooperative territory defence and digging out shelters, but not by alloparental brood care, which only benefits the breeding group members. In our study, dominant female reproduction was not affected by relatedness to the subordinate female. Neither the number of clutches laid nor clutch size and egg mass differed between the treatments ( Fig. 2e , Supplementary Fig. S3 ). This is consistent with predictions from a recent model of pay-to-stay suggesting that subordinates should only compensate for the costs they inflict on dominant reproduction, but not provide net fitness benefits to dominants in excess of this contribution [28] . Consequently, the genetic fitness of dominants should be largely independent of the degree of relatedness to subordinate helpers and hence their reproductive decisions should be unaffected by kinship. In contrast, helping to gain indirect benefits predicts that dominant females should base their reproductive effort on the degree of relatedness to their helpers: If kin-selection is primarily responsible for cooperation among the group members, related subordinates should be more helpful than unrelated ones, which would allow adaptive adjustment of reproduction of dominant females [51] . In contrast to the lack of a kinship effect on reproduction of dominant females, subordinate female reproduction was affected by relatedness to the dominant female, namely with regard to egg mass: subordinate females unrelated to the dominant female laid smaller eggs than related ones. Two main, non-mutually exclusive hypotheses could explain this effect. First, female–female competition may have been more severe in the non-kin than in the kin treatment, and the dominants’ coercion of unrelated females to provide help apparently has raised their alloparental brood care effort and, consequently energy expenditure [36] . In addition, coercion of dominants might have increased stress in subordinate females. Experimental manipulation of stress levels in this species has suggested that stressed N. pulcher females produce smaller eggs [52] , which is consistent with this interpretation and in turn supports the conclusion that coercion may explain increased helping in this experiment. However, we did not find strong indications that female–female aggression depended on kinship ( Supplementary Fig. S2 and Supplementary Table S1 ). Second, subordinates could be selected to increase reproductive effort if their offspring enjoy a higher survival probability due to relatedness with the dominant female (for example, if brood cannibalism is contingent on relatedness to the brood). The latter explanation also fits the brood care pattern observed for subordinate female clutches. Subordinate females provided more maternal brood care in the non-kin treatment, which might serve as a defence against egg cannibalism by the dominant female. Alternatively, this increase in maternal brood care could reflect a behavioural compensation for the observed small egg size of unrelated helpers. To our knowledge this is the first study testing for kinship effects on reproduction experimentally in a cooperatively breeding vertebrate, therefore comparisons with other species are presently not possible. Our study generally confirms that kinship is an important component in cooperative systems, but remarkably relatedness may have effects contrary to predictions from conventional kin-selection theory, if coercion by dominants is involved. It is important to note here that group augmentation is likely to generate fitness benefits of helping in this species as well [24] , [48] , but due to our experimental design this mechanism cannot explain the differences found between the experimental treatments in this study. Rather, dominants and unrelated subordinates seem to trade different commodities reciprocally against each other, thereby generating fitness benefits to both. Animals N. pulcher ( Fig. 1 ) is endemic to Lake Tanganyika and breeds cooperatively in groups of a dominant pair and typically 1 to 25 subordinates of different size classes [24] , [53] , [54] . Kin recognition has been demonstrated [55] and both related and unrelated subordinates participate in brood care of dominants’ broods by cleaning and fanning the eggs [19] , in territory defence against predators, space competitors and conspecific intruders [19] , [29] , [53] , [54] , and in territory maintenance (for example, digging out shelters [47] , [53] ). The social conditions in this species seem to predispose it to the operation of some sort of trading help against resource access, such as assumed in evolutionary pay-to-stay models [26] , [27] , [28] : overall relatedness is low [16] , [42] and subordinates impose costs on the dominants by reducing the growth of the dominant female [40] and by occasional participation in reproduction [40] , [49] . Furthermore, predation risk is the major environmental factor constraining dispersal [19] , [48] , and individuals are long-lived, reaching 3 years of age or more [34] . For a comprehensive review of cooperative breeding in N. pulcher see ref. 39 . Experimental set-up We used captive descendants from N. pulcher individuals caught in the wild in 1996 and 2006 (Lake Tanganyika near Kasakalawe point, Zambia). They were measured, sexed and kept singly shortly before the experiment. Experimental groups were established of a pair and a subordinate female in a 100-l compartment of a 400-l tank subdivided by opaque partitions (in total, eleven 400-l tanks were used; Supplementary Fig. S1 ). The bottom of the aquarium was covered with a layer of sand ( ∼ 3 cm). Each experimental compartment contained two clay flower pot halves serving as breeding substrate, two translucent tubes suspended near the surface to serve as refuge and a suspended filter. Each group contained a male that was unrelated to both females, ensuring that subordinate females in the kin treatment and in the non-kin treatment had similar incentives to mate with the dominant male and to inherit the territory. By restricting this experiment to female subordinates we avoided potential problems arising from sex-specific dispersal strategies. Like in nature [54] , in each group the dominant male was the largest individual (mean: 63.2 mm body length (BL), range: 33.5–88.0), followed by the dominant female (mean: 49.9 mm BL, range: 25.6–68.9) and the subordinate female (mean: 35.7 mm BL, range: 22.0–60.3). The degree of relatedness was experimentally varied between the subordinate female and the dominant female, with half of the groups containing related females (sisters or daughters: r =0.5) and the other half containing unrelated females ( r =0.0; Supplementary Fig. S1 ). The groups were assembled following a standardized protocol: First the subordinate female was released and allowed to acclimatize to the new territory for 24 h. Then both pair members were released. If the subordinate female was evicted from her group, the experiment was terminated after 46 days, or in some cases earlier to prevent injury of the subordinate. Thereafter, the group was replaced by a new group of the same treatment. We obtained a total sample size of 69 groups ( n =33 non-kin and 36 kin treatment groups). Recording of evictions Subordinate female eviction was first checked 1 h after release of the dominants, and subsequently once a day for the whole experimental duration. We categorized eviction on an ordinal scale as: ‘accepted’ when the subordinate was allowed to visit the breeding shelter without being attacked and chased away by dominants; ‘tolerated’ when the subordinate moved freely in the compartment including the bottom area were the breeding pair usually spends most of the time, but when it was attacked and chased away if closely approaching the breeding shelter; ‘evicted’ when the subordinate was hiding behind or in the refuges (filters or suspended bottles) in the top part of the compartment, and when it was attacked when moving out of its refuge. Brood care and reproduction Brood care was observed and quantified following a protocol established in previous studies [35] , [40] . The frequencies of egg cleaning acts and egg fanning bouts were recorded during a 15-min observation period for both females and the male. Besides direct brood we also recorded indirect brood care, specifically the frequency of carrying sand out of the brood cavity (digging). The clutch was assigned to the dominant or the subordinate female using observations of sham-spawning and substrate cleaning behaviour of the breeding shelter on the days preceding clutch deposition. This method has been validated by molecular parentage analysis and was shown to yield very little error [35] . After the brood care observation the eggs were temporarily removed, counted and a sample of ∼ 5 eggs was collected for egg mass assessment. The pot was returned within 10 min and all the fish resumed brood care after this disturbance. The removed eggs were dried for 36 h at 70 °C and the average single-egg dry-mass was determined (total dried egg mass/number of eggs: abbreviated ‘egg mass’ throughout) using a scale (Mettler-Toledo, 0.01 mg accuracy). A few clutches did not allow brood care observation and egg mass determination, and as a result sample sizes may vary slightly for these analyses. Compensation experiment After a dominant female had produced the third clutch, we assigned this group randomly to a clutch size reduction treatment (later referred to as reduction treatment) or to a control treatment. In both treatments we used a cylindrical netting wire to fence off the breeding pair for 10 min. During these 10 min only the helper female was inside the netting wire and hence had access to the brood cavity with the eggs. The netting wire allowed the breeding pair to see into the area with the brood cavities, but it prevented them from entering. In the reduction treatment we then temporarily removed the clutch, scraped-off half of the eggs, placed back the remaining eggs and fed 5–10 of the scraped-off eggs to the helper female. In the control treatment we only removed 1 to 5 eggs (maximum 10% of the total number of eggs, for determining the egg mass) and also placed back the clutch. Subsequently we removed the netting wire and the group could again move freely in the entire tank. One hour after the manipulation we conducted a brood care observation, following the brood care observation protocol described above (post-treatment brood care). We repeated this manipulation during three consecutive clutches (clutch 3 to 5) and then switched to the other treatment (clutch 6 to 8) for each group separately. Our aim was that the dominant breeders perceive this clutch size reduction by 50% in the reduced treatment as a result of brood cannibalism by the helper [56] , thereby we simulated a significant cost of the helper presence to the pair. We expected that helpers should compensate for this cost by increasing their alloparental brood care subsequently, and predicted a significantly stronger effect on the behaviour of unrelated helpers. Behavioural data One hour after release of the pair we conducted a 15 min focal observation of each group, recording the frequencies of restrained and overt aggression and submission of all the group members, and the frequencies of subordinate female visits inside the breeding shelters. Statistical analyses All analyses where conducted using SPSS 17.0. We used an ordinal regression with logit-link to analyse subordinate female eviction. Sample sizes were n =36 kin and n =33 non-kin in each model. The difference in body size between the dominant male and the subordinate female (ordinal regression, P =0.70) and the body size of the subordinate female (ordinal regression, P =0.12) were not significant when entered into the model containing the difference between the body sizes of the two females. Female body size is a confounding factor in N. pulcher reproduction and (allo)parental brood care and female–female interactions [35] , and was, therefore, statistically controlled for throughout the paper. The numbers of dominant and subordinate clutches produced were analysed using separate GLM with a log-link, adding the observation period of each group as a covariate. Dominant and subordinate clutch sizes and brood care were analysed using separate general estimating equation models, again with a log-link (entering individual identifiers as subjects to account for repeated measures per individual female). Similarly, we used two general estimating equations with identity-link to analyse egg mass of dominant and subordinate females separately. In all models we used the deviance method for adjusting parameter scaling, and entered kin treatment (kin or non-kin) as a factor and female body size as a covariate. For the brood care observations we also added clutch size as a covariate. For all analyses the number of individuals ( N ); and additionally for repeated measures the number of clutches is given ( n ). Submission, aggression and breeding substrate visits were analysed using GLM with a log-link assuming poisson distribution. Nonsignificant interactions (notably, kinship × size difference in females within a group were invariably nonsignificant P >0.70, GLM) were not included in the final model. D.H. came up with the idea and designed the experiment together with M.Z. and M.T. M.Z., D.H., N.C. performed the experiment and D.H. analysed the data. M.Z. and M.T. wrote the paper. How to cite this article: Zöttl, M. et al . Kinship reduces alloparental care in cooperative cichlids where helpers pay-to-stay. Nat. Commun. 4:1341 doi: 10.1038/ncomms2344 (2013).